Exact controllability of complex networks Controlling complex networks is of paramount importance in science and engineering. Despite the recent development of structural controllability theory, we continue to lack a framework to control undirected complex networks, especially given link weights. Here we introduce an exact controllability paradigm based on the maximum multiplicity to identify the minimum set of driver nodes required to achieve full control of networks with arbitrary structures and link-weight distributions. The framework reproduces the structural controllability of directed networks characterized by structural matrices. We explore the controllability of a large number of real and model networks, finding that dense networks with identical weights are difficult to be controlled. An efficient and accurate tool is offered to assess the controllability of large sparse and dense networks. The exact controllability framework enables a comprehensive understanding of the impact of network properties on controllability, a fundamental problem towards our ultimate control of complex systems. One of the most challenging problems in modern network science and engineering is controlling complex networks. Although great effort has been devoted to understanding the interplay between complex networks and dynamical processes taking place on them [1] , [2] , [3] , [4] , [5] in various natural and technological systems [6] , [7] , [8] , [9] , [10] , [11] , [12] , [13] , [14] , [15] , [16] , the control of complex dynamical networks remains to be an outstanding problem. Generally, because of the ubiquity of nonlinearity in nature, one must consider the control of complex networked systems with nonlinear dynamics. However, at present there is no general framework to address this problem because of the extremely complicated interplay between network topology and nonlinear dynamical processes, despite the development of nonlinear control [17] , [18] , [19] , [20] , [21] , [22] in certain particular situations such as consensus [23] , communication [24] , [25] , traffic [26] and device networks [17] , [27] . To ultimately develop a framework to control complex and nonlinear networks, a necessary and fundamental step is to investigate the controllability of complex networks with linear dynamics. There exist well developed theoretical frameworks of controllability for linear dynamical systems in the traditional field of engineering control [28] , [29] , [30] , [31] , [32] . However, significant challenges arise when applying the traditional controllability framework to complex networks [33] because of the difficulty to determine the minimum number of controllers. A ground-breaking recent contribution was made by Liu et al . [34] who developed a minimum input theory to efficiently characterize the structural controllability of directed networks, allowing a minimum set of driver nodes to be identified to achieve full control. In particular, the structural controllability of a directed network can be mapped into the problem of maximum matching [35] , [36] , [37] , where external control is necessary for every unmatched node. The structural controllability framework also allows several basic issues to be addressed, such as linear edge dynamics [38] , lower and upper bounds of energy required for control [39] , control centrality [40] and optimization [41] . Although the structural controllability theory offers a general tool to control directed networks, a universal framework for exploring the controllability of complex networks with arbitrary structures and configurations of link weights is lacking. Mathematically, the framework of structural controllability is applicable to directed networks characterized by structural matrices, in which all links are represented by independent free parameters [34] . This requirement may be violated if exact link weights are given, motivating us to pursue an alternative framework beyond the structural controllability theory. For undirected networks, the symmetric characteristic of the network matrix accounts for the violation of the assumption of structural matrix, even with random weights. Thus, we continue to lack a reliable tool to measure the controllability of undirected networks. For some practical issue concerning actual control, such as predicting the control energy with given link weights, necessary and sufficient conditions to ensure full control are the prerequisite. Taken together, we need a more general and accurate framework to study the controllability of complex networks. In this paper, we develop an exact controllability framework as an alternative to the structural controllability framework, which offers a universal tool to treat the controllability of complex networks with arbitrary structures and link weights, including directed, undirected, weighted and unweighted networks with or without self-loops. Structural controllability can be reproduced by our framework for structural matrix that can be ensured by assigning random weights to directed links. In particular, based on the Popov–Belevitch–Hautus (PBH) rank condition [42] that is equivalent to the Kalman rank condition [28] , we prove that the minimum number of independent driver nodes or external controllers is equal to the maximum geometric multiplicity of all eigenvalues of the network matrix. If the network matrix is diagonalizable, for example, as for undirected networks, controllability is simply determined by the maximum algebraic multiplicity of all eigenvalues; that is, the minimum number of inputs is determined by the dimension of eigenvectors for arbitrary networks and, for symmetric networks, this number is nothing but the eigenvalue degeneracy. For simple regular networks, their exact controllability can be calculated analytically. For more complicated model networks and many real-world weighted networks with distinct node-degree distributions, the exact controllability can be efficiently assessed by numerical computations. The minimum set of driver nodes can be identified by elementary transformations based on the exact controllability framework. A systematic comparison study indicates that the results from our exact controllability theory are consistent with those in ref. 34 for cases where both frameworks are applicable. Application of our framework also reveals a number of phenomena that cannot be uncovered by the structural controllability framework. For example, we find that for random [43] and small-world networks [6] , [44] with identical link weights, the measure of controllability is a non-monotonic function of the link density with the largest controllability occurring in the intermediate region. For highly sparse or dense networks, the former being ubiquitous in real-world systems, the exact controllability theory can be greatly simplified, leading to an efficient computational paradigm in terms solely of the rank of matrix. Exact controllability measurement of complex networks A necessary step towards ultimately controlling nonlinear network systems is to fully understand the controllability of complex networks with linear dynamics. Consider a network of N nodes described by the following set of ordinary differential equations: where the vector x =( x 1 , ⋯ , x N ) T stands for the states of nodes, A ε R N × N denotes the coupling matrix of the system, in which a ij represents the weight of a directed link from node j to i (for undirected networks, a ij = a ji ). u is the vector of m controllers: u =( u 1 , u 2 , ⋯ , u m ) T , and B is the N × m control matrix. The classic Kalman rank condition [28] , [45] stipulates that system (equation (1)) can be controlled from any initial state to any final state in finite time if and only if rank( C 1 )=rank[ B , AB , A 2 B ,..., A N −1 B ]= N . The standard way to address the controllability problem is to find a suitable control matrix B consisting of a minimum number of driver nodes so as to satisfy the Kalman rank condition. However, a practical difficulty is that there are 2 N possible combinations of the driver nodes. The notion of structural controllability was then introduced by Lin [29] and was recently adopted to directed complex networks [34] . Relying on the maximum matching algorithm, the structural controllability framework developed by Liu et al . [34] enables efficiently identifying a minimum set of unmatched nodes that need to be controlled to achieve full control of the system. Thus, the unmatched nodes are the driver nodes, the number of which determines the controllability of the network. The computation complexity of finding B based on the efficient maximum matching algorithm can therefore be significantly reduced. In general, the structural controllability theory is valid for directed networks associated with structural matrices in which all links are represented by independent free parameters. This limitation prompts us to develop an exact controllability framework for arbitrary network structures and link weights. To formulate a theoretical framework of exact controllability, we need a new starting point. Our theory is based on the PBH rank condition [32] , [42] , [45] , [46] from control theory, according to which system (equation (1)) is fully controllable if and only if is satisfied for any complex number c , where I N is the identity matrix of dimension N . It can be proved that, if and only if any eigenvalue λ belonging to matrix A satisfies equation (2), full control can be ensured [32] , [42] , [45] , [46] . For system (equation (1)), there are many possible control matrices B that satisfy the controllable condition. The central goal is to find a set of B corresponding to the minimum number N D of independent drivers or controllers required to control the whole network. In general, N D is defined in terms of B as N D =min{rank( B )}, as in the structural controllability-based formulation [34] . The PBH condition has been employed recently to study the controllability of leader–follower systems [47] and regular graphs [48] , [49] . We develop a general theory to calculate N D based on the PBH rank condition (see Methods and Supplementary Note 1 ). It can be proven that for arbitrary network structures and link weights, say arbitrary matrix A , the minimum number N D of controllers or drivers is determined by the maximum geometric multiplicity μ ( λ i ) of the eigenvalue λ i of A : where μ ( λ i )= dim V λ i = N −rank( λ i I N − A ) and λ i ( i =1,..., l ) represents the distinct eigenvalues of A . For undirected networks with arbitrary link weights, N D is determined by the maximum algebraic multiplicity δ ( λ i ) of λ i : where δ ( λ i ) is also the eigenvalue degeneracy of matrix A . We need to stress that equation (3) is rigorous and generally valid without any limitations for matrix A and equation (4) is proven to be valid for general undirected networks with diagonalizable matrix A . To compute the geometric and algebraic multiplicities for large networks is computationally demanding. However, the task can be greatly simplified if the network is either sparse or dense. In fact, complex networks arising in real-world applications are typically sparse [1] . For a large sparse network, in which the number of links scales with N in the limit of large N [50] , with a small fraction of self-loops, N D is simply determined by the rank of A : For a densely connected network with identical link weights w , in which the zeros in A scale with N in the limit of large N , with a small fraction of self-loops, we have With the simplified formulas (equation (5)) and (equation (6)), N D can be evaluated by computing the rank of the network matrix A or wI N + A in an efficient manner. For undirected sparse networks, LU (lower and upper matrix) decomposition with computation complexity O ( N 2.376 ) [51] can yield reliable results of rank( A ). For other types of networks, (singular-value decomposition) method with O ( N 3 ) [52] can give accurate results of rank( A ) as well as the eigenvalues of A . The measure of controllability n D , or simply controllability, of a network can be defined as the ratio of N D to the network size N [34] : Identify driver nodes We offer a general approach to identifying a minimum set of driver nodes that need to be controlled by using the PBH rank condition (equation (2)). According to the exact controllability theory, N D is determined by the maximum geometric multiplicity μ ( λ M ) of the eigenvalue λ M . Thus, the control matrix B to ensure full control should satisfy the condition (equation (2)) by substituting λ M for the complex number c , as follows: The question becomes how to find the minimum set of drivers identified in B to satisfy equation (8). We note that the rank of the matrix [ λ M I N − A , B ] is contributed by the number of linearly independent rows. In this regard, we implement elementary column transformation on the matrix λ M I N − A (or A − λ M I N ), which yields a set of linearly dependent rows that violate the full rank condition (equation (8)). The controllers located via B should be imposed on the identified rows to eliminate all linear correlations to ensure condition (equation (8)). The nodes corresponding to the linearly dependent rows are the drivers with number N −rank( λ M I N − A ), which is nothing but the maximum geometric multiplicity μ ( λ M ). Note that each column in B can at most eliminate one linear correlation, such that the minimum number of columns of B , say, min{rank( B )} is the same as the number μ ( λ M ) of drivers, regaining our exact controllability theory. To illustrate the method explicitly, we present three typical simple examples, as shown in Fig. 1 . For each graph, we first compute the eigenvalues λ of the matrix A and their geometric multiplicity μ ( λ ) to find the eigenvalue λ M corresponding to the maximum geometric multiplicity μ ( λ M ). The matrix A − λ M I N associated with λ M can then be established so as to identify linear correlations. We perform elementary column transformation on A − λ M I N to obtain its column canonical form that reveals the linear dependence among rows. The rows that are linearly dependent on other rows correspond to the driver nodes that need to be controlled to maintain full control. Note that the configuration of drivers is not unique as it depends on the order of implementing the elementary transformation and there are many possible choices of linearly dependent rows. Nevertheless, the minimum number of drivers is fixed and determined by μ ( λ M ), analogous to the structural controllability theory. The approach of finding drivers is rigorous, ensured by the PBH rank condition, the maximum multiplicity theory (MMT) and the column canonical form associated with matrix rank. Thus, the method is applicable to arbitrary networks, including networks described by structural matrices. We have tested its performance on structural matrix by assigning each link a random parameter, which shows excellent agreement with the result from the structural controllability framework ( Supplementary Fig. S1 and Supplementary Note 2 ), but with different computational efficiency. The maximum matching algorithm with computation complexity O ( N 1/2 L ; L denotes the number of links) outperforms our elementary transformation-based algorithm with O ( N 2 (log N ) 2 ) (ref. 53 ) for dealing with structural matrices. 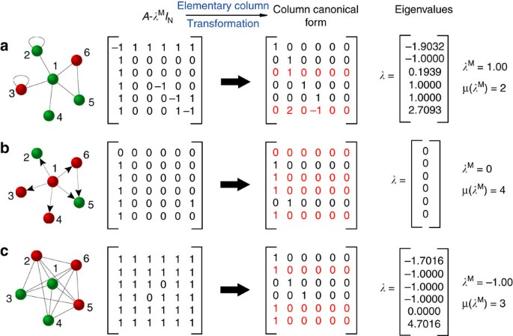Figure 1: Illustration of the exact controllability framework to identify a minimum set of drivers. (a) A simple undirected network with self-loops, (b) a simple directed network and (c) an undirected network with dense connections. The matrixA−λMIN, the column canonical form of matrixA−λMINby the elementary column transformation, the eigenvaluesλand the eigenvalueλMcorresponding to the maximum geometric multiplicityμ(λM) ofAare given for each simple network. The rows that are linearly dependent on others in the column canonical form are marked by red. The nodes corresponding to them are the drivers that are marked by red as well in the networks. For the undirected networks inaandc,μ(λM) is equal to the maximum algebraic multiplicity, that is, the multiplicity ofλM. The configuration of drivers is not unique as it relies on the elementary column transformation, but the number of drivers is fixed and determined by the maximum geometric multiplicityμ(λM) of matrixA. Figure 1: Illustration of the exact controllability framework to identify a minimum set of drivers. ( a ) A simple undirected network with self-loops, ( b ) a simple directed network and ( c ) an undirected network with dense connections. The matrix A − λ M I N , the column canonical form of matrix A − λ M I N by the elementary column transformation, the eigenvalues λ and the eigenvalue λ M corresponding to the maximum geometric multiplicity μ ( λ M ) of A are given for each simple network. The rows that are linearly dependent on others in the column canonical form are marked by red. The nodes corresponding to them are the drivers that are marked by red as well in the networks. For the undirected networks in a and c , μ ( λ M ) is equal to the maximum algebraic multiplicity, that is, the multiplicity of λ M . The configuration of drivers is not unique as it relies on the elementary column transformation, but the number of drivers is fixed and determined by the maximum geometric multiplicity μ ( λ M ) of matrix A . Full size image In general, our framework of exact controllability can quantify the minimum number of drivers and identify them. Applying the framework to model and real networks will provide deep insights into the significant problem of network control. Exact controllability of model and real networks We now present controllability measure n D of a large number of model networks with identical- and random-weight distributions and real-world unweighted and weighted networks from the exact controllability theory and the structural controllability theory in cases where it is applicable. In many real situations, it is not possible to have the exact link weights because of the measurement noise and nonlinear effects. Thus, it is reasonable to assume random-weight distributions rather than identical weights when dealing with real networks. However, in some man-made networks, identical weights or a small number of different weights are possible, prompting us to consider the controllability of unweighted networks. Further, revealing the effect of network topology on a variety of dynamics is of paramount theoretical importance in network science and with tremendous interest [1] , [2] , [3] . As the central issue related to network dynamics, the influence of topology on controllability deserves to be fully understood in unweighted networks without complications from other factors. Considered together, we study n D with respect to unweighted networks (identical weights) and networks with random weights. For undirected regular graphs with identical weights, N D and the relevant eigenvalues can be calculated precisely, as listed in Table 1 . We see that the chain and ring graphs can be controlled by one and two controllers, respectively. However, for the star and fully connected networks, almost all nodes need to be independently controlled. The results of chain and star networks are consistent with those from the structural controllability theory [34] , but the results of ring and fully connected networks are different ( Supplementary Note 3 ). This difference, as will be explained below, indicates the need for the exact controllability framework. Table 1 Eigenvalues and minimum number of driver nodes of regular unweighted, undirected graphs. 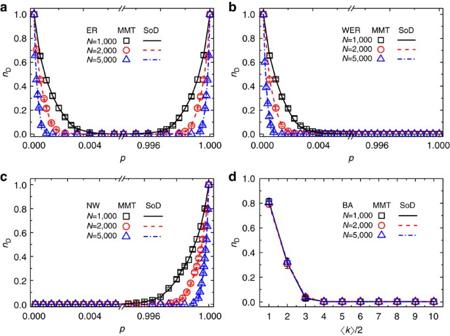Figure 2: Exact controllability of undirected networks. Exact controllability measurenDas a function of the connecting probabilitypfor (a) unweighted ER random networks and (b) ER random networks with random weights assigned to links (WER). (c)nDversus the probabilitypof randomly adding links for Newman–Watts small-world networks. (d)nDversus half of the average degree ‹k›/2 for Barabási–Albert scale-free networks. All the networks are undirected and their coupling matrices are symmetric. The data points are obtained from the MMT equation (4) and the error bars denote the s.d., each from 20 independent realizations. The curves (SoD) are the theoretical predictions of equations (5) and (6) for sparse and dense networks, respectively. The representative network sizes used areN=1,000, 2,000 and 5,000. Full size table Figure 2a shows, for Erdös–Rényi (ER) random networks [43] with identical link weights, the controllability measure n D as a function of the connecting probability p . We see that, regardless of the network size, for small values of p (for example, p <0.006), n D decreases with p . However, for high link density (for example, p -values exceeding 0.994), n D begins to increase towards ( N −1)/ N , which is exact for p =1. This counterintuitive increase in n D was not noticed before our work, but our exact controllability theory reveals that it can be attributed to the impact of identical link weights. Note that n D is symmetric about p =0.5, which can be qualitatively explained by the density function of the eigenvalues of random matrices [54] : Figure 2: Exact controllability of undirected networks. Exact controllability measure n D as a function of the connecting probability p for ( a ) unweighted ER random networks and ( b ) ER random networks with random weights assigned to links (WER). ( c ) n D versus the probability p of randomly adding links for Newman–Watts small-world networks. ( d ) n D versus half of the average degree ‹ k ›/2 for Barabási–Albert scale-free networks. All the networks are undirected and their coupling matrices are symmetric. The data points are obtained from the MMT equation (4) and the error bars denote the s.d., each from 20 independent realizations. The curves (SoD) are the theoretical predictions of equations (5) and (6) for sparse and dense networks, respectively. The representative network sizes used are N =1,000, 2,000 and 5,000. Full size image which is a continuous function. As the multiplicity measure is discrete, ρ ( λ ) cannot be used to derive n D . Nonetheless, the positive correlation between the peak of ρ ( λ ) and the maximum multiplicity can be exploited to explain the behaviour of n D . In particular, the maximum of ρ ( λ ) occurs at [54] , which is symmetric about p =0.5, in agreement with the behaviour of n D , providing an explanation for the symmetry of n D about p =0.5. Figure 2b shows the behavior n D for undirected ER random networks [43] with random link weights. We see that n D is a decreasing function of p and the increasing behaviour in n D in the region of high link density disappears. Figure 2c,d show the results for undirected small-world and scale-free networks in the absence of weights (or with identical link weights), respectively. We see that the value of n D for Newman–Watts small-world networks [44] is 2/ N for zero probability p of randomly adding edges but n D quickly reduces to 1/ N as p increases from zero and remains at the value of 1/ N until p exceeds a large value, for example, 0.994, after which n D increases towards ( N −1)/ N . Such behaviours are analogous to those for the ER random network. The reason that n D is close to the value of 2/ N for p =0 can be attributed to the fact that the Newman–Watts small-world networks are constructed from a ring-like network for which N D =2 holds. Figure 2d shows, for Barabási–Albert scale-free networks [7] of different values of the average degree ‹ k ›, the behaviour of n D . We observe that, for small values of ‹ k ›, n D displays the same decreasing trend as for random networks. 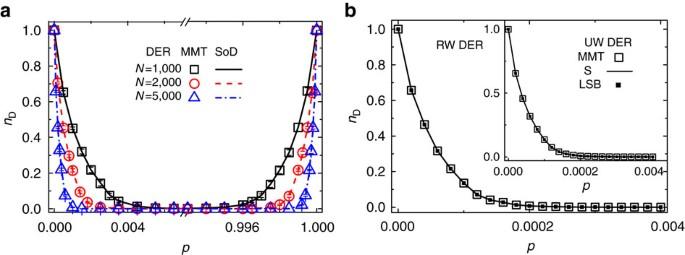Figure 3: Exact controllability of directed networks. (a) Exact controllability measurenDas a function of connecting probabilitypin directed ER random networks with identical weights (DER) for different network sizes. (b) Exact controllability and structural controllabilitynDversuspin directed ER random networks with random weights (RW DER) in the absence of bidirectional links. The inset ofb, exact controllability and structural controllabilitynDversuspin unweighted, directed ER random networks (UW DER) in the absence of bidirectional links. Here MMT stands for the exact controllability determined by the maximum geometric multiplicity equation (3), SoD stands for the exact controllability of sparse or dense networks from equations (5) and (6), respectively, S denotes the exact controllability of sparse networks from equation (5) and, LSB denotes the structural controllability from the maximum matching algorithm. Ina,andare in good agreement with each other for different network sizes. Inb,,andcoincide exactly without any difference in the network described by the structural matrix. In the inset ofb, the assumption of structural controllability is weakly violated, ascribed to the unweighted property of the network. The structural controllabilityis still consistent with the exact controllabilitybut with negligible difference. For example, atp=8 × 10−4,=0.21584, whereas=0.21576. Atp=10−3,=0.1352, whereas=0.1350. For the networks ina, the connecting probabilities of two directions between two nodes are bothp, but the corresponding random variables are independent of each other. For the networks inb, based on the structure of an undirected ER random network, we randomly assign a direction to each undirected link. All the results are from 20 independent realizations and the error bars denote the s.d. The network size inbis 5,000. Figure 3 shows the controllability n D of directed networks with identical and random weights, where the latter in the absence of bidirectional links can be exactly addressed by the structural controllability framework. In Fig. 3a , the behaviors of n D of directed ER random networks with identical weights and possible bidirectional links are somewhat similar to those of their undirected counterparts. Thus, high demand of drivers and controllers in dense networks holds for any network structures with identical link weights. In Fig. 3b , a random weight is assigned to each directed link, resulting in a structural matrix, allowing the comparison between the exact and the structural controllability. The assumption of structural matrix is ensured by the random weights together with the directed structure. We find the behaviors of n D resulting from both methods are in complete agreement with each other, indicating the reduction of the exact controllability theory to the structural controllability for structural matrix. We have also tested the difference between the two theories if the assumption of structural matrix is weakly violated by setting identical weights, as shown in the inset of Fig. 3b . We observe consistent results with negligible difference from each other, suggesting the applicability of the structural controllability in directed sparse networks with given link weights and the insensitivity of controllability to the link weights in sparse networks. Figure 3: Exact controllability of directed networks. ( a ) Exact controllability measure n D as a function of connecting probability p in directed ER random networks with identical weights (DER) for different network sizes. ( b ) Exact controllability and structural controllability n D versus p in directed ER random networks with random weights (RW DER) in the absence of bidirectional links. The inset of b , exact controllability and structural controllability n D versus p in unweighted, directed ER random networks (UW DER) in the absence of bidirectional links. Here MMT stands for the exact controllability determined by the maximum geometric multiplicity equation (3), SoD stands for the exact controllability of sparse or dense networks from equations (5) and (6), respectively, S denotes the exact controllability of sparse networks from equation (5) and, LSB denotes the structural controllability from the maximum matching algorithm. In a , and are in good agreement with each other for different network sizes. In b , , and coincide exactly without any difference in the network described by the structural matrix. In the inset of b , the assumption of structural controllability is weakly violated, ascribed to the unweighted property of the network. The structural controllability is still consistent with the exact controllability but with negligible difference. For example, at p =8 × 10 −4 , =0.21584, whereas =0.21576. At p =10 −3 , =0.1352, whereas =0.1350. For the networks in a , the connecting probabilities of two directions between two nodes are both p , but the corresponding random variables are independent of each other. For the networks in b , based on the structure of an undirected ER random network, we randomly assign a direction to each undirected link. All the results are from 20 independent realizations and the error bars denote the s.d. The network size in b is 5,000. Full size image We have also found that the exact controllability of undirected and directed networks with identical weights can be estimated by the cavity method [36] , [37] developed for studying structural controllability, offering a good analytical prediction and revealing the underlying relationship between the structural controllability and the exact controllability ( Supplementary Fig. S2 and Supplementary Note 4 ). Tables 2 and 3 display, respectively, the exact controllability measure of a number of real-directed and -weighted networks. In both Tables, and stand for the result from our exact controllability and simplified theory (equation (5)), respectively. From Table 2 , we see that the values of agree with those of for all real networks, owing to the fact that these real-world networks are sparse. For Table 2 , as the networks are directed, the structural controllability measure, denoted by , can also be calculated. For all cases except the food webs, the values of and are quite close. In general, we observe the inequality . The consistency between the results from our exact controllability theory and from the structural controllability theory confirms the similarity between them for directed and unweighted networks. Further validation of our theory is obtained by assigning random weights to all the networks in Table 2 . In this case, the coupling matrices of all networks become structural matrix, and the new values of are exactly the same as the values of for the networks associated with structural matrices. For the originally weighted real-world networks, only the values of and are given, as shown in Table 3 . Table 2 Exact controllability measures of real unweighted, directed networks. Full size table Table 3 Exact controllability measures of real-weighted networks. Full size table We have developed a maximum multiplicity theory to characterize, exactly, the network controllability in terms of the minimum number of required controllers and independent driver nodes. Our approach by transforming the network controllability problem into an eigenvalue problem greatly facilitates analysis and offers a more complete understanding of the network controllability in terms of extensive existing knowledge of network spectral properties. Our theory is applicable to any network structures, directed or undirected, with or without link weights and self-loops. Our exact controllability framework can reproduce the structural controllability for directed networks associated with structural matrices. For dense or sparse networks, our theory can be simplified, resulting in formulas that can be used to calculate the minimum number of driver nodes in an efficient manner. This is particularly encouraging, as most real-world complex networks are sparse. We have studied a large number of real-world networks and compared with the results predicted by the structural controllability theory in cases where it is applicable. Despite the advantage of our theory in studying the controllability of complex networks, insofar as the exact weights of links are unknown, at the present the structural controllability framework is still the best approach to evaluating the controllability of directed networks. This is mainly because of its error-free characteristic based on the maximum matching algorithm. In contrast, our framework relies on the eigenvalues and the rank of the network matrix, the evaluation of which inevitably contains numerical errors, although such error can be controlled by high-accurate algorithms, such as the SVD algorithm. In addition, the structural controllability approach outperforms our method in terms of the computational efficiency in identifying the minimum set of drivers. For example, in our method, finding driver nodes based on the elementary transformation requires time on the order of O ( N 2 (log N ) 2 ), whereas the structural controllability framework requires time on the order of O ( N 1/2 L ) to find unmatched nodes, where L is the total number of links. Nevertheless, our exact controllability framework can have a broader scope of applications. For example, if the weights of partial links are available, the framework will offer better measurement of the controllability by setting the weights of other unavailable links to be random parameters, namely, partial structural matrix. Our framework is also valid for undirected networks, where the structural matrix assumption is slightly violated because of the network symmetry. The framework is as well applicable to networks containing a number of self-loops with identical or distinct weights, which will have quite different consequences. Further, exploring exact controllability is important to achieving actual control and predicting control energy, especially in man-made networks. Taken together, our exact controllability theory as an alternative to the structural controllability theory offers deeper understanding of our ability to control complex networked systems. Exact controllability measurement for general networks For an arbitrary matrix A in system (equation (1)), there exists an N × N nonsingular matrix P such that A = PJP −1 or P −1 AP = J with J =diag( J ( λ 1 ), J ( λ 2 ), ⋯ , J ( λ l )), where λ i ( i =1,..., l ) represents the distinct eigenvalues of A and J ( λ i ) is the Jordan block matrix of A associated with λ i [55] . For every distinct eigenvalue λ i of matrix A , there are two concepts of multiplicity [55] . (i) Algebraic multiplicity δ (λ i ): multiplicity of eigenvalue λ i , which satisfies , where δ ( λ i ) is also the eigenvalue degeneracy; (ii) geometric multiplicity μ ( λ i ): the dimension of the eigenspace of A associated with λ i , that is, μ ( λ i )= dim V λ i = N −rank( λ i I N − A ). Note that the geometric multiplicity is determined by the eigenvectors associated with the eigenvalues, which means that both multiplicities depend on the eigenvalues of the matrix A . In general, we have μ ( λ i ) ⩽ δ ( λ i ). The two types of multiplicities will be used to derive our theory of exact controllability. According to the definition of μ ( λ i ), we can find that μ ( λ i ) is equal to the number of the basic Jordan blocks in J ( λ i ) [55] , that is, J ( λ i )=diag( j 1 , j 2 , ⋯ , j μ ( λ i ) ), where j s ( s =1,2, ⋯ , μ ( λ i )) is the basic Jordan block matrix having the form exemplified by equation (11) below. The key to our theory lies in bridging the two multiplicities and the controllability via the PBH rank condition [42] . Applying the nonsingular transformation y = P −1 x and Q = P −1 B , we can rewrite system (equation (1)) in Jordan form as It can be verified that systems (equation (1)) and (equation (10)) have the same controllability in the sense that rank( λI N − A , B )=rank( λI N − J , Q ), with rank( B )=rank( Q ). We call Q the transformed control matrix, which can be used to calculate the control energy ( Supplementary Note 5 ). Any basic Jordan block matrix j ( λ ) associated with eigenvalue λ has the form: For each j ( λ ) of order v , all elements in the first column of matrix λI v − J are zero and other v −1 columns are independent of each other. We thus have rank( λI v − j ( λ ))= v −1. As the number of basic Jordan blocks associated with eigenvalue λ i is equal to its geometric multiplicity μ ( λ i ), the number of zero columns in λ i I N − j ( λ ) is μ ( λ i ) and other N − μ ( λ i ) columns are independent of each other, yielding rank( λ i I N − J )= N − μ ( λ i ). The PBH rank condition [42] stipulates that system (equation (1)) is controllable if and only if for each λ i of matrix A , the following holds: Because of the rank inequality [56] , equation (12) can be rewritten as N =rank( λ i I N − J , Q ) ⩽ rank( λ i I N − J )+rank( Q ) so that rank( Q )≥ N −rank( λ i I N − J ). Recalling that rank( Q )=rank( B ), we have Equation (13) will be satisfied if rank( B ) is larger than or equal to the maximum value of N −rank( λ i I N − J ) for all eigenvalues λ i . It can be shown that the equality in equation (13) can be satisfied by specific construction of Q , indicating the necessity of establishing Q via nonsingular transformation associated with the Jordan blocks ( Supplementary Note 2 ). In this regard, the minimum value of rank( B ) is the maximum value of N −rank(λ i I N − J ); that is, the minimum number N D of independent driver nodes, min{rank( B )}, is max i { N −rank( λ i I N − J )}. As this is equivalent to max i { N −rank( λ i I N − A )}, according to the definition of geometric multiplicity, we have equation (3): N D =max i { μ ( λ i )}. Although the maximum geometric multiplicity as the lower bound of the number of controllers has been implied in linear control theory [32] , [46] and some literature [47] , [48] , [49] , we prove that the maximum multiplicity is both necessary and sufficient conditions to ensure full control and offer a rigorous scheme to identify the minimum set of drivers, leading to the development of an exact and efficient controllability framework. If A is diagonalizable, for example, for undirected networks, then we have μ ( λ i )= δ ( λ i ) for each eigenvalue and the number of independent drivers or controllers under this condition is determined by equation (4): N D =max i { δ ( λ i )}. Our theory thus offers an exact characterization of the controllability of complex networks with any structures and weights in the presence or absence of self-loops. It should be emphasized that N D =max i { δ ( λ i )} is valid for undirected network or diagonalizable matrix A . In addition, we can show that the observability of complex networks can be formulated in a similar way ( Supplementary Note 6 ). Exact controllability for dense and sparse networks For a large sparse network in the absence of self-loops, the expectation of eigenvalues of the coupling matrix A is ; therefore, the maximum geometric multiplicity occurs at the eigenvalue λ =0 with high probability [57] . Moreover, it can be proven that the geometric multiplicity associated with the zero eigenvalue is equal to the rank deficiency [56] : μ (0)= N −rank( A ). The minimum number of controllers and independent drivers as determined by the geometric multiplicity associated with the zero eigenvalue can then be estimated by equation (5): N D =max{1, N −rank( A )}. For a densely connected network with unit link weights, the zeros in A scales with N in the limit of large N . In the absence of loops, the probability is high to find two groups of nodes that are interconnected and have mutual neighbours. In general, in this case the coupling matrix consists of many rows of the form The corresponding rows in det( λI N − A ) of the characteristic polynomial are We see that if λ =−1, the two rows are identical. We then have [54] det(− I N − A )=det( I N + A )=0. As a result, −1 is the eigenvalue of the matrix (equation (14)). As, in a dense network with unit weights, the likelihood to observe two rows with the form in matrix (equation (14)) is high, λ =−1 becomes the eigenvalue corresponding to the maximum multiplicity, enabling an efficient formulation of exact controllability for dense networks. In particular, the geometric multiplicity is defined as N −rank(λ i I N − A ). Substituting λ by −1 yields N D =max{1, N −rank( I N + A )}. For identical link weights of arbitrary value w , the eigenvalue becomes − w rather than −1. Substituting λ by − w yields equation (6): N D =max{1, N −rank( wI N + A )}. Equations (5) and (6) are the exact controllability theory for any sparse networks and dense networks with identical link weights, respectively. It is noteworthy that, although we assume the absence of self-loops so as to derive the simplified formulas (equation (5)) and (equation (6)), they are still valid in the presence of a small fraction of self-loops, insofar as the self-loops do not violate the dominations of 0 and − w in the eigenvalue spectrum of matrix A for sparse and dense networks, respectively. In fact, the combination of the number and the weight distribution of self-loops has quite intricate roles in the controllability, which will be discussed thoroughly elsewhere. Computation of matrix rank and eigenvalues We use the SVD method [52] to compute the eigenvalues of matrix A of any complex networks required by the general MMT for quantifying the exact controllability of complex networks. To count the number of eigenvalues with the same value, that is, the algebraic multiplicity, we set a small threshold 10 −8 . If the absolute difference between two eigenvalues is less than the threshold, they are regarded as identical. We have checked that the maximum algebraic multiplicity is quite robust to the setting of the threshold. This is because of the fact that this multiplicity usually arises at integer eigenvalues that are independent of the threshold. The SVD method can also be used to calculate the accurate rank of the matrix associated with an arbitrary network. For sparse networks and dense networks with identical weights, the exact controllability is only determined by the rank of the matrix. For sparse, undirected networks with identical or random weights, we have checked that the LU decomposition method [51] can yield reliable results of the matrix rank, in good agreement with those from the SVD method. However, for other types of networks, we have to rely on the SVD method. For both LU and SVD methods, the tolerance level is set to be 10 −8 . If a value in the diagonal is less than the threshold, it will be treated as zero to determine the matrix rank. We have examined that the matrix rank is insensitive to the threshold insofar as it is sufficiently small. All the exact controllability measures of real networks presented in Tables 2 and 3 are obtained via the SVD method to ensure accuracy. The structural controllability of networks is computed via the maximum matching algorithm [34] . For the elementary column transformation for identifying driver nodes, we use the Gaussian elimination method with computation complexity O ( N 2 (log N ) 2 ) (ref. 53 ) to obtain the column canonical form that reveals the linear dependence among rows. How to cite this article: Yuan, Z. et al . Exact controllability of complex networks. Nat. Commun. 4:2447 doi: 10.1038/ncomms3447 (2013).